Vibrational coherence probes the mechanism of ultrafast electron transfer in polymer–fullerene blends The conversion of photoexcitations into charge carriers in organic solar cells is facilitated by the dissociation of excitons at the donor/acceptor interface. The ultrafast timescale of charge separation demands sophisticated theoretical models and raises questions about the role of coherence in the charge-transfer mechanism. Here, we apply two-dimensional electronic spectroscopy to study the electron transfer process in poly(3-hexylthiophene)/PCBM (P3HT/PCBM) blends. We report dynamics maps showing the pathways of charge transfer that clearly expose the significance of hot electron transfer. During this ultrafast electron transfer, vibrational coherence is directly transferred from the P3HT exciton to the P3HT hole polaron in the crystalline domain. This result reveals that the exciton converts to a hole with a similar spatial extent on a timescale far exceeding other photophysical dynamics including vibrational relaxation. Organic solar cells use a blend of electron donating materials, such as conjugated polymers and electron accepting materials, typically [6,6]-phenyl-C 61 butyric acid methyl ester (PCBM) to convert light energy to electrical energy. A question in this field has been how the electron–hole binding energy is overcome to generate mobile carriers and the photovoltaic effect [1] , [2] , [3] , [4] , [5] . Recent developments show that the electron and hole are not as firmly bound as basic arguments suggest [6] , [7] , [8] . Relevant work includes reports that mobile carriers are rapidly produced by hot-exciton dissociation [6] . In other words, excitation at energies higher than the optical gap may be an important route for dissociation of the bound electron–hole pair. Nevertheless, Salleo and co-workers [9] clearly demonstrated that photocurrent is just as effectively generated (in terms of quantum efficiency) when exciting well to the low-energy side of the band gap as compared with exciting to the high-energy side. That work suggests that at equilibrium the charge carriers tend to be separated, not bound. To elucidate the mechanism of charge separation in more detail, new techniques have been developed to directly probe the dynamics of mobile carriers. The diffusion of uncorrelated charge carriers was monitored by Gulbinas et al . [10] , [11] Beard and co-workers [12] show that mobile carriers are efficiently photogenerated. Recently, Heeger and co-workers [13] have pointed out a curious trend that exciton dissociation in donor–acceptor blends is remarkably fast—they speculate that it does not require exciton migration to an interface. Friend and co-workers [7] examined the ultrafast dissociation of excitons using a Stark probe and did indeed detect exceptionally fast charge separation. Charges apparently can separate to 4 nm in the time span of only 40 fs. The ultrafast timescale of charge separation demands theoretical models that go beyond equilibrium theories like Marcus theory and furthermore raises questions about coherence and the role of non-equilibrium nuclear configurations. It is important in this regard for the experiment to provide incisive information about charge separation dynamics that helps to shape and test theoretical models. To elucidate information about electron transfer pathways that will guide theory more rigorously, we turn to two-dimensional electronic spectroscopy (2D ES). 2D ES inherently has both high time and frequency resolution and has been used to elucidate the photo-initiated dynamics in complex condensed-phase systems [14] , [15] . 2D ES is very similar to one-dimenisonal pump–probe, in which molecules are excited and a spectrum of excited states, as well as their population dynamics along pump–probe delay time axis are recorded. 2D ES differs from one-dimenisonal pump–probe by simultaneously labelling each state by their energies on the excitation axis. Thus, a 2D ‘map’ is obtained with information encoding real-time correlations between energies of states photoexcited and states probed [16] . Here, we apply 2D ES to investigate the process of ultrafast exciton dissociation in model donor–acceptor heterostructures. The 2D ES ‘map’, that enables direct detection of hot carrier formation [17] and vibrational coherence ‘labelling’ helps provide insights into the mechanism for charge separation [18] , in particular the properties of the photogenerated hole. In this work, we perform 2D ES measurements to study ultrafast electron transfer dynamics in P3HT/PCBM blends. We use a laser pulse, compressed to ~11 fs ( Supplementary Fig. 1 and Supplementary Note 1 ) and centred at ~600 nm with a spectral width sufficiently broad to excite the lowest two vibronic peaks of P3HT aggregates (semicrystalline domain) and simultaneously probe the tail of P3HT-hole absorption, Fig. 1b . Films tend to scatter and are prone to photodegradation [19] , so here we instead study model nanoparticle (NP) heterostructures formed by flash co-precipitating regioregular poly(3-hexylthiophene-2,5-diyl) (P3HT), of molecular weight 50–70 kDa, with 10 or 20 wt% PCBM [20] . As comparison, we also report studies on neat P3HT NPs. 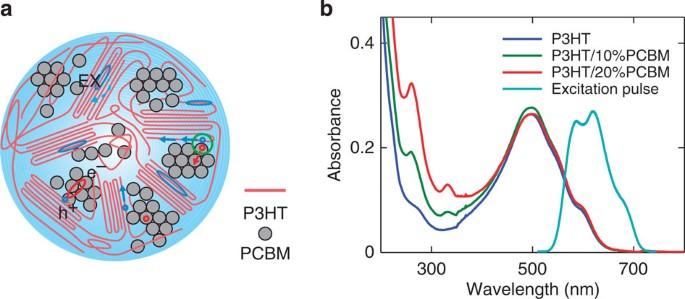Figure 1: Polymer–fullerene heterostructure NPs. (a) Schematic illustration of P3HT/PCBM-blended NP structure: light blue ellipses represent excitons; light blue circles and red circles/ellipse represent holes and electrons, respectively; blue and red arrows represent the direction of hole and electron motion, respectively; the green circle represents a bound electron–hole pair. (b) absorption spectra of neat P3HT, P3HT/10%PCBM, P3HT/20%PCBM NP aqueous suspensions and excitation pulse spectrum. Figure 1: Polymer–fullerene heterostructure NPs. ( a ) Schematic illustration of P3HT/PCBM-blended NP structure: light blue ellipses represent excitons; light blue circles and red circles/ellipse represent holes and electrons, respectively; blue and red arrows represent the direction of hole and electron motion, respectively; the green circle represents a bound electron–hole pair. ( b ) absorption spectra of neat P3HT, P3HT/10%PCBM, P3HT/20%PCBM NP aqueous suspensions and excitation pulse spectrum. Full size image NP structure and steady-state absorption P3HT/PCBM NPs have been characterized in previous work [20] . Transmission electron microscopy ( Supplementary Fig. 2 and Supplementary Note 2 ) shows that NPs have a diameter of ~20–50 nm. A schematic structural model of the P3HT/PCBM NPs is displayed in Fig. 1a . The folded P3HT chains form a 2D plane that further stack into lamellae [21] . PCBM molecules either form crystallites or are dispersed within amorphous domains of P3HT. Figure 1b shows the absorption spectra of P3HT NP and P3HT/PCBM NP aqueous suspensions. The spectrum of neat P3HT NP from 350 to 640 nm is fit using a linear combination of the monomer absorption spectrum ( Supplementary Fig. 3 and Supplementary Note 3 ) and a series of Gaussian functions, which account for the vibronic progression of P3HT aggregates. Two shoulders appearing at 604 and 556 nm correspond to 0–0 and 0–1 transitions, respectively, of P3HT aggregates [22] , [23] . These transitions provide evidence that the NPs have characteristics similar to films. The presence of PCBM in the P3HT/PCBM NPs is evident by the absorption bands at 260 and 340 nm. 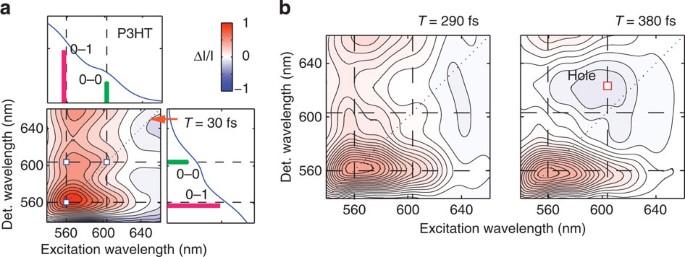Figure 2: Representative absorptive 2D electronic spectra of neat P3HT NP aqueous suspensions. (a) 2D spectra of neat P3HT NP at 30 fs along with linear absorption spectrum. Green and red bars label peak positions corresponding to 0–0 and 0–1 transitions obtained from fitting the linear absorption spectrum. Dashed lines are used as guides for peak positions. In the 2D spectra, the peak corresponding to the 0–1 transition is slightly shifted relative to 556 nm due to the convolution of the excitation pulse and molecular response functions. (b) 2D spectra of neat P3HT NP at 290 and 380 fs. The PIA is attributed to the absorption of P3HT hole polarons. Photoexcited dynamics in neat P3HT NPs Figure 2 displays representative absorptive 2D spectra of a neat P3HT NP aqueous suspension at different waiting times (pump–probe delay times), together with the linear absorption spectrum to illustrate peak positions. Two positive peaks at 560 and 604 nm along the diagonal correspond to 0–1 and 0–0 vibronic bands of the P3HT crystalline domain. Since these two transitions have a common ground state, there appear two cross peaks with exciting (detecting) wavelength and detecting (exciting) wavelength at 560 and 604 nm, respectively. Downhill energy transfer due to vibrational relaxation causes the amplitude of the upper cross peak to increase as a function of the waiting time. The overall decay of the 0–1 exciton population occurs with a time constant of 241 fs (analysis reported in Supplementary Table 1 , Supplementary Fig. 4 and Supplementary Note 4 ). Figure 2: Representative absorptive 2D electronic spectra of neat P3HT NP aqueous suspensions. ( a ) 2D spectra of neat P3HT NP at 30 fs along with linear absorption spectrum. Green and red bars label peak positions corresponding to 0–0 and 0–1 transitions obtained from fitting the linear absorption spectrum. Dashed lines are used as guides for peak positions. In the 2D spectra, the peak corresponding to the 0–1 transition is slightly shifted relative to 556 nm due to the convolution of the excitation pulse and molecular response functions. ( b ) 2D spectra of neat P3HT NP at 290 and 380 fs. The PIA is attributed to the absorption of P3HT hole polarons. Full size image At a waiting time of 380 fs, a broad negative-going feature, with exciting wavelength at 604 nm and detecting wavelength centred at ~620 nm, is clearly seen in the 2D spectrum. This feature is assigned to photoinduced absorption (PIA) of holes generated in P3HT domains on the basis of previous studies by Vardeny and coworkers [24] , [25] . These authors [25] used PIA-detected magnetic resonance spectroscopy to confirm the assignment of this peak. They showed that this peak, with associated infrared-active vibrational modes, corresponds to a spin-1/2 state. The interpretation of this feature in terms of the hole polaron absorption is further supported by more recent work [26] , [27] , [28] , [29] , [30] (including our current work). Specifically, the amplitude of this feature increases in magnitude with the addition of a small amount of PCBM, as will be discussed further below, suggesting the dissociation of excitons and subsequent formation of hole polarons. These results indicate that this peak corresponds to the product of exciton dissociation in P3HT domain, that is, hole polaron. We exclude the possibility of thermal modulation [31] on the PIA signal in our experiment on the basis that the thermal modulation of P3HT should occur on much longer timescales and is outside of the spectral window of the present analysis (the thermal artifact overlaps the ground-state bleaching (GSB) signal, that is, 560 and 604 nm peak). Thus, we attribute the PIA cross peak to the hole-polaron absorption. Stimulated emission (SE) appearing as cross peaks with detecting wavelength above 640 nm is also observed within 100 fs ( Supplementary Fig. 5 ). The observation of SE on this timescale is consistent with ultrafast broadband photoluminescence measurements by Hodgkiss and coworkers [32] . The SE partially overlaps the PIA cross peak, which gives rise to the relatively ‘narrow’ band of the PIA observed in the neat P3HT NPs. Hole-polaron formation in neat P3HT films has been observed on the timescale of hundreds of femtoseconds by pump–probe in previous reports [25] , [28] . Silva and coworkers [33] suggested that exciton dissociation may occur in neat P3HT films at the interface between ordered and disordered domains. Rumbles and coworkers [21] verified this point by performing time-resolved microwave conductivity measurements on films with different microstructures. Two mechanisms have been proposed for the polaron formation in neat conjugated polymer films: hot-exciton dissociation and thermalized exciton dissociation [34] . Ito and coworkers [35] found that when exciting at 400 nm, hot-exciton dissociation occured within ~100 fs. In our experiment in which only the lowest two vibronic states (the 0–0 and 0–1 transitions) of P3HT aggregates are photoexcited, we observe that the PIA of hole polarons appears at 380 fs. This result suggests that exciton relaxation precedes exciton dissociation in neat P3HT NPs for the excitation conditions that we have used in these experiments. Ultrafast dynamics and coherence in P3HT/PCBM blends Representative 2D spectra of P3HT/10%PCBM NP and P3HT/20%PCBM NP aqueous suspensions at different waiting times are displayed in Fig. 3a,b , respectively. In contrast to the neat P3HT NP aqueous suspension, the PIA of P3HT hole in the P3HT/PCBM blend NPs appears very rapidly—it is clearly evident in these data when comparing the relative amplitude of the bleach and PIA at a waiting time as rapid as 35 fs. The amplitude of the PIA feature appears somewhat larger in P3HT/20%PCBM when compared with P3HT/10%PCBM, consistent with a larger fraction of excitons dissociating with a higher fullerene loading. The PIA from the hole obscures the cross-peak bleach as well as the 0–0 diagonal feature at 600 nm in these datasets. 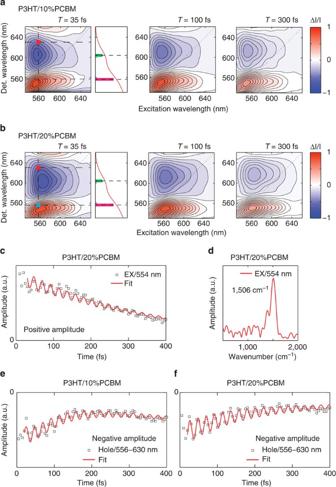Figure 3: Absorptive 2D spectra and time traces of P3HT/PCBM NP aqueous suspensions. (a,b) 2D spectra of P3HT/10%PCBM and P3HT/20%PCBM, respectively, at 35, 100 and 300 fs, together with linear absorption to illustrate peak positions. Red and blue squares are guides for the peak positions of time traces in fig. (c,e,f). (c) Representative time trace of diagonal peak with exciting and detecting wavelengths both at 554 nm for P3HT/20%PCBM NPs. The trace is fit with the sum of a constant background, monoexponential function and exponentially damped-cosine function. The amplitude modulations oscillate with a period of ~20 fs. The amplitude modulation is attributed to vibrational coherence of C=C stretching mode. (d) Fourier transformation of oscillatory term, which gives a peak at ~1,506 cm−1. (e,f) Time traces of PIA with exciting wavelength at 556 nm and detecting wavelength at 630 nm for both P3HT/10%PCBM and P3HT/20%PCBM blends. These two time traces are fit with a sum of constant background, two/three exponential functions and exponentially damped-cosine function (shown inSupplementary Tables 2 and 3). Vibrational coherences due to the C=C stretching mode are also observed in the PIA. Figure 3: Absorptive 2D spectra and time traces of P3HT/PCBM NP aqueous suspensions. ( a , b ) 2D spectra of P3HT/10%PCBM and P3HT/20%PCBM, respectively, at 35, 100 and 300 fs, together with linear absorption to illustrate peak positions. Red and blue squares are guides for the peak positions of time traces in fig. ( c , e , f ). ( c ) Representative time trace of diagonal peak with exciting and detecting wavelengths both at 554 nm for P3HT/20%PCBM NPs. The trace is fit with the sum of a constant background, monoexponential function and exponentially damped-cosine function. The amplitude modulations oscillate with a period of ~20 fs. The amplitude modulation is attributed to vibrational coherence of C=C stretching mode. ( d ) Fourier transformation of oscillatory term, which gives a peak at ~1,506 cm −1 . ( e , f ) Time traces of PIA with exciting wavelength at 556 nm and detecting wavelength at 630 nm for both P3HT/10%PCBM and P3HT/20%PCBM blends. These two time traces are fit with a sum of constant background, two/three exponential functions and exponentially damped-cosine function (shown in Supplementary Tables 2 and 3 ). Vibrational coherences due to the C=C stretching mode are also observed in the PIA. Full size image The rapid appearance of the PIA suggests hot-exciton dissociation competes with vibrational relaxation in the excited electronic state of P3HT aggregates in P3HT/PCBM blends. To see whether the exciton is likely to be vibrationally hot during the fast exciton dissociation process, we analysed the vibrational–relaxation dynamics in P3HT/PCBM blends. In Fig. 3c , we plot the amplitude of the diagonal peak corresponding to 0–1 transition in the P3HT/20%PCBM sample. An exponential fit to the amplitude as a function of the waiting time reveals that the exciton population decays with a time constant of 310 fs—so vibrational relaxation is much slower than electron transfer. We compare vibrational–relaxation dynamics with the time dependence of the hole polaron PIA. Figure 3e,f display time traces of PIA with exciting wavelength at 556 nm and detecting wavelength at 630 nm of P3HT/PCBM blends. The latter represents the tail of the hole absorption and is selected to examine the dynamics since this position has least overlap with the positive cross peak corresponding to GSB signal. The time traces are fit by using a nonlinear least square method: the fit function consists of a sum of two/three exponential functions, a damped-cosine function and a constant background. The fitting results are listed in Supplementary Tables 2 and 3 . 2D ES spectra of both P3HT/PCBM blends show similar dynamical evolution. The cross-peak contains overlapping signal contributions—the positive-signed GSB and, the dominant, negative-signed hole PIA. The early-time dynamics show an increase in magnitude of the PIA contribution (that is, the cross-peak becomes more negative) with a time constant of ~24 fs (analysis reported in Supplementary Tables 2 and 3 , Supplementary Fig. 4 and Supplementary Note 4 ). This is indicative of the formation of hole polarons through hot electron transfer. The magnitude of the PIA then diminishes (that is, the cross-peak becomes less negative) with a time constant of ~150 fs for P3HT/20%PCBM. This likely stems from the growth of the positive-signed bleach cross-peak as a result of vibrational relaxation ( cf. the time constant 241 fs of the decay of diagonal peak in the neat P3HT NP). The PIA then further increases in magnitude (that is, the cross-peak becomes more negative) on a longer timescale—this observation likely arising from the dissociation of thermalized excitons. These results therefore suggest that the fastest electron transfer is facilitated by hot-exciton dissociation. The 0–1 bleach amplitude oscillates strongly with a period of ~20 fs. Fourier transformation with respect to the waiting-time axis gives a frequency of ~1,506±40 cm −1 ( Fig. 3d ). This value corresponds to the energy difference between the 0–0 and 0–1 vibronic transitions that we coherently excited. It is the C=C stretching mode, as suggested by Raman spectroscopy [36] . The dephasing time of this vibrational coherence was found to be ~250 fs by fitting the time trace. We also observe vibrational coherence with the same oscillation frequency in the hole polaron PIA cross-peak ( Fig. 3e,f ). The hole polaron is generated through exciton dissociation; therefore, the observation of coherence in the hole polaron PIA suggests that the oscillations of the bleach on the diagonal can, at least partially, be attributed to vibrational coherence in the excited electronic state. A fit to the time trace gives a dephasing time ~230 fs. The oscillating PIA is photogenerated by coherent excitation of the 0–0 and 0–1 P3HT bands and is detected as a cross-peak. In the event that exciton relaxation (an incoherent process) precedes electron transfer, the coherence is expected to be absent. Since the coherence is retained in the PIA amplitude, the P3HT exciton must be able to dissociate from either vibronic state of the P3HT exciton. Hence, the retention of vibrational coherence during electron transfer provides firm evidence for hot-exciton dissociation. Hot-exciton dissociation indicates that electron transfer precedes vibrational relaxation and the electron transfer reaction occurs in a non-equilibrium state, that is, nuclear configuration and charge distribution are not in equilibrium. In organic photovoltaics, both vibrational relaxation of the C=C stretching mode and electron transfer are considered as fast processes (on the timescale of hundreds of femtosecond) [37] . However, no explicit time constant has been reported for the vibrational relaxation in neat conjugated polymers. Recent studies of hot-exciton photoluminescence/fluorescence upconversion show that vibrational cooling occurs on the timescale of hundreds of femtoseconds [32] , [38] . This is consistent with our observation in neat P3HT NPs. In P3HT/PCBM blends, we show that the hole polaron population rises with a time constant of ~24 fs. By comparing neat P3HT and P3HT/PCBM NPs, we conclude that electron transfer occurs through the dissociation of hot excitons in P3HT/PCBM blends. It is not possible to directly link our observation of ultrafast electron transfer from both vibronic states to the overall device efficiency since the overall device efficiency is determined by photoexcited dynamics, including exciton diffusion, electron transfer, charge separation, charge recombination, charge collection and so on. Salleo and coworkers [9] found that the internal quantum efficiency (IQE) in the P3HT/PCBM-based device is wavelength independent. Their result indicates that hot electron transfer is not required for device performance. This is true especially in systems with large electron transfer driving force because electron transfer from both ‘hot’ and relaxed excited states can be very efficient in such systems. However, hot electron transfer might still play an important role for charge separation in system with low electron transfer driving force. For example, Lanzani and coworkers [6] reported that a delocalized charge-transfer state, generated by hot electron transfer could effectively contribute to free carriers generation and lead to a gain in IQE. Our present study does not provide information about the role of hot electron transfer on device efficiency. Our result also indicates that the vibrational wavepacket generated by femtosecond broadband excitation of P3HT exciton in the crystalline domain modulates the amplitude of the product, that is, hole-polaron PIA in P3HT. There are two possible implications. One is that the vibrational coherence modulates the reaction coordinate (or the electron transfer rate) and the product is formed periodically [39] , [40] . The other mechanism is that the vibrational coherence is not strongly coupled to the reaction coordinate [41] . So the C=C stretching mode is a spectator mode that is carried along with the reaction [41] , [42] . However, a recent experimental study [43] of coherent nuclear wavepacket evolution shows that the vibrational mode involving large displacement of carbon atoms in the backbone is strongly coupled to the charge-transfer reaction. Detailed calculation of ultrafast charge transfer in an oligothiophene–fullerene heterojunction supports the likelihood that the sustained coherence of the vibrational wavepacket is related to electronic coherence in the ultrafast charge transfer [44] . Recently, Falke et al . [45] probed the coherence in a different spectral window from 440 to 530 nm and reported the coherence observed in PCBM following electron transfer. However, in our work, we directly observe coherence in both excitonic peaks and polaronic peaks in P3HT domain. In this spectral region, it is anticipated that contributions from the electron acceptor are very small as the relative oscillator strength in this spectral region is strongly biased towards P3HT. We show that the vibrational coherence photogenerated with P3HT exciton is retained in P3HT domain through the electron transfer process and can be used as a probe to reveal the charge-transfer mechanism from the perspective of the electron donor. The study reported here shows how vibrational coherence is an excellent way to tag the initial superposition of states and follow their evolution. It is quite surprising that the vibrational wavepacket is faithfully retained from the exciton to the photogenerated hole in the crystalline P3HT domain. It confirms that the exciton dissociates by electron transfer to the fullerene domain. The strong amplitude of the vibrational coherence in the PIA also indicates that the photogenerated hole exhibits either the same extent of the delocalization as the P3HT exciton, or is more localized, because delocalization diminishes the Huang–Rhys factor via ‘exchange narrowing’. Finally, it is interesting that ‘hot’ electron transfer is so prevalent in the P3HT–PCBM aggregates. The fast electron transfer from both vibronic states suggests that the driving force for electron transfer derives from the strong coupling between the directly photoexcited singlet states and high-lying charge-transfer states, rather than a single favourable acceptor electron affinity. Sample preparation and linear absorption P3HT NP and P3HT/PCBM (with weight percent: 10%PCBM+90%P3HT, 20%PCBM+80%P3HT) NP aqueous suspensions were prepared as described previously [20] . The solutions were filtered by 0.45 μm nonsterile nylon syringe filters to remove the large particulates. The sample is characterized by transmission electron microscopy ( Supplementary Note 2 ). The ultraviolet–visible absorption spectra were measured by a Cary 300 Bio UV–vis (Varian) spectrometer. The absorption spectra of all samples were measured before and after experiments and no more than 2% change was observed, indicating that the NPs were stable to photo-oxidation and precipitation. Ultrafast spectroscopy The 2D ES setup is described in detail elsewhere [46] . Briefly, a 150 fs, 800 nm laser pulse, generated by a 5 kHz regenerative amplifier (Spitfire Pro, Spectra-Physics), was used to produce a broadband laser pulse by a home-built NOPA. The laser pulse had a spectral width ~74 THz, centred at about 600 nm and was compressed to ~11 fs via a combination of a grating compressor and a prism compressor. The FROG of the excitation laser pulse is displayed in Supplementary Fig. 1 . The compressed pulse then hit a 2D diffractive optic and generated four first-order diffraction beams, arranged in a BOXCARS configuration. The four beams crossed at the sample position. The energy of the laser pulse that was used to excite the sample was 8 nJ per pulse. A third-order signal, generated in the background free direction interfered with an attenuated beam (termed as ‘local oscillator’). The interference pattern was detected by a CCD camera (Andor, Newton). Three pairs of silica wedges controlled the time delays between three excitation pulses. The time delay ( t 1 ) between the first two pulses was scanned from −45 to 45 fs, with a 0.2-fs step. The Fourier transformation along t 1 axis generated excitation frequency (or wavelength) axis. The dynamics were monitored by scanning pump–probe delay time axis (waiting time— t 2 , the time delay between the second pulse and third pulse) from 0 to 400 fs with a 5-fs step. The phasing of the 2D spectra was achieved by using the projection-slice theorem [47] , with the pump–probe measurement performed under the same experimental conditions as the 2D experiment. We determined the phase for these 2D measurements by using a standard reference sample (cresyl violet perchlorate ethanol solution). Pump–probe and 2D spectra of cresyl violet percholorate were obtained under the same experimental condition as the 2D ES of P3HT (P3HT/PCBM) NP; the phase parameter obtained from analysis of the dye data was subsequently applied to the polymer (polymer/fullerene) NP datasets. Power dependence study was reported in Supplementary Fig. 6 and Supplementary Note 5 . Data were analyzed by using MATLAB. How to cite this article: Song, Y. et al . Vibrational coherence probes the mechanism of ultrafast electron transfer in polymer–fullerene blends. Nat. Commun. 5:4933 doi: 10.1038/ncomms5933 (2014).